Role of biogenic silica in the removal of iron from the Antarctic seas Iron has a key role in controlling biological production in the Southern Ocean, yet the mechanisms regulating iron availability in this and other ocean regions are not completely understood. Here, based on analysis of living phytoplankton in the coastal seas of West Antarctica, we present a new pathway for iron removal from marine systems involving structural incorporation of reduced, organic iron into biogenic silica. Export of iron incorporated into biogenic silica may represent a substantial unaccounted loss of iron from marine systems. For example, in the Ross Sea, burial of iron incorporated into biogenic silica is conservatively estimated as 11 μmol m −2 per year, which is in the same range as the major bioavailable iron inputs to this region. As a major sink of bioavailable iron, incorporation of iron into biogenic silica may shift microbial population structure towards taxa with relatively lower iron requirements, and may reduce ecosystem productivity and associated carbon sequestration. Siliceous phytoplankton are abundant and productive components of marine ecosystems, with diatoms accounting for ~43% of annual marine carbon fixation worldwide [1] . Sedimentation of the dense silica produced by these microorganisms has a critical role in the transport of carbon to the deep ocean [2] and may also enhance the export of phosphorus and nitrogen below the mixed layer [3] , [4] . Previous observations of iron in siliceous frustules of cultured diatoms [5] suggests that sedimentation of biogenic silica may also be a quantitatively significant mechanism for the removal of bioavailable iron. Yet, this potential mechanism has remained largely unexplored in natural settings. Diatoms often dominate phytoplankton communities in seasonally ice-covered Antarctic coastal seas, such as the Ross Sea [6] . Primary production and microbial community composition in this region are variably limited by a number of physical conditions and nutrients, including iron [7] , [8] , [9] , which in turn affects biological carbon dioxide uptake and therefore climate [6] . Although these waters are the most productive regions of the Southern Ocean [10] and major sites of atmospheric carbon dioxide uptake [11] , the mechanisms governing the cycling of the limiting nutrient iron are not well understood in these [8] and other ocean areas. On the basis of this gap in knowledge, combined with renewed interest in iron fertilization as an approach to the current climate crisis [12] , an improved understanding of iron cycling in marine systems is critical. Building on studies in which total iron quotas of single cells were quantified [13] , we present both the content and speciation of iron contained in one biological pool relatively less subject to remineralization: iron incorporated into biogenic silica. We show this pool represents a significant iron removal mechanism from Ross Sea surface waters. Chemical treatments Diatoms of the genus Fragilariopsis dominated the community of siliceous plankton sampled along a transect of the Western Antarctic coastal ocean, followed by silicoflagellates. Subsets of these specimens were chemically treated with trace metal grade reagents to isolate the pool of iron incorporated into silica. These treatments included washes with 6 N hydrochloric acid, which removed organic coatings and loosely associated iron, or 30% hydrogen peroxide, which targeted organic iron material on the silica surface [14] . Sixty-six individual specimens (17 untreated, 26 peroxide washed and 23 acid washed) were analysed using X-ray fluorescence (XRF) microscopy and X-ray absorption near edge structure (XANES) spectroscopy. Iron morphology XRF micrographs of single specimens revealed two morphologically distinct forms of iron: (1) iron that mirrored silicon distributions and (2) occasional micron-sized regions of high iron content (termed hotspots) ( Fig. 1 ). The per-pixel iron content of the former correlated strongly with per-pixel silicon content in each specimen, confirming structural incorporation of iron into biogenic silica ( Fig. 2 ). This pattern was much unlike the distribution of other trace metals, such as manganese, which appeared to be surface associated ( Fig. 2 ). 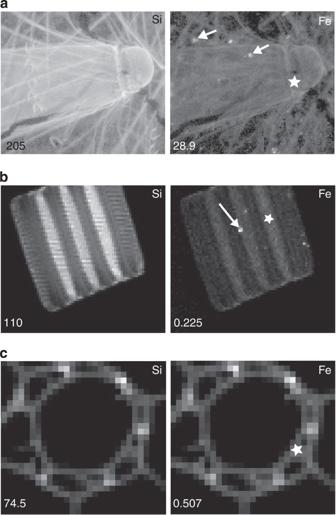Figure 1: XRF micrographs. Maps of iron (Fe) and silicon (Si) content in siliceous specimens, includingCorethronspp. (a),Fragilariopsisspp. (b) and silicoflagellates (c) revealed two morphologically distinct iron pools associated with biogenic silica: iron colocalizing with silica (stars) and micron-sized iron hotspots (arrows). Stars and arrows indicate regions that were further investigated with iron XANES. The number in the lower left corner of each image is the maximum elemental content (μg cm−2) represented by white (elemental content scales linearly, with black as zero). The heights of images in rowsa,bandcare 66, 27 and 26 μm, respectively. All images were collected from untreated samples (that is, no peroxide or acid treatment). Figure 1: XRF micrographs. Maps of iron (Fe) and silicon (Si) content in siliceous specimens, including Corethron spp. ( a ), Fragilariopsis spp. ( b ) and silicoflagellates ( c ) revealed two morphologically distinct iron pools associated with biogenic silica: iron colocalizing with silica (stars) and micron-sized iron hotspots (arrows). Stars and arrows indicate regions that were further investigated with iron XANES. The number in the lower left corner of each image is the maximum elemental content (μg cm −2 ) represented by white (elemental content scales linearly, with black as zero). The heights of images in rows a , b and c are 66, 27 and 26 μm, respectively. All images were collected from untreated samples (that is, no peroxide or acid treatment). 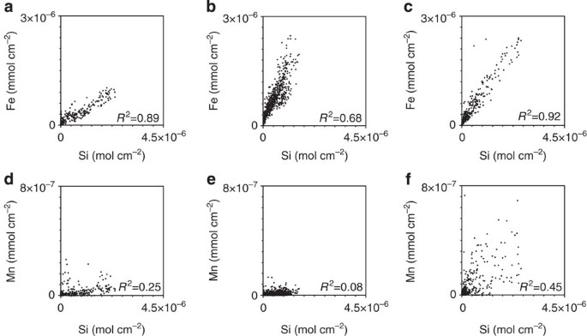Figure 2: Scatter plots of elemental content. Typical data collected from three individual specimens ofFragilariopsisspp. (such as those inFig. 1b) are displayed as scatter plots of per-pixel elemental content. In all specimens, the pool of iron (Fe) that colocalized with silicon (Si), that is, excluding hotspots, correlated positively with silicon content (a–c). This pattern is consistent with structural incorporation of iron, as thicker areas of silicon correspond to a proportionally higher content of iron. In contrast, manganese (Mn) is typically associated with particles, such as biogenic silica, as a surface coating. Consistent with this surface distribution, Mn content did not exhibit a relationship with Si content (d–f). Scatter plots in each column were generated from the same single specimen. All plots were generated from untreated samples (that is, no peroxide or acid treatment). Full size image Figure 2: Scatter plots of elemental content. Typical data collected from three individual specimens of Fragilariopsis spp. (such as those in Fig. 1b ) are displayed as scatter plots of per-pixel elemental content. In all specimens, the pool of iron (Fe) that colocalized with silicon (Si), that is, excluding hotspots, correlated positively with silicon content ( a – c ). This pattern is consistent with structural incorporation of iron, as thicker areas of silicon correspond to a proportionally higher content of iron. In contrast, manganese (Mn) is typically associated with particles, such as biogenic silica, as a surface coating. Consistent with this surface distribution, Mn content did not exhibit a relationship with Si content ( d – f ). Scatter plots in each column were generated from the same single specimen. All plots were generated from untreated samples (that is, no peroxide or acid treatment). Full size image Iron speciation Several lines of evidence generated from the XANES analysis demonstrate that iron incorporated into biogenic silica is reduced and likely present in organic form. First, the average XANES spectrum of iron incorporated into silica exhibited a K-edge position that was substantially lower than that of the average iron hotspot by 2.8±0.3 eV ( Fig. 3 ). This lower K-edge is consistent with a reduced oxidation state of iron in the biogenic silica. Second, the position of the pre-edge centroid, another strong indicator of iron oxidation state [15] , revealed a continuum of oxidation states, with incorporated iron being more reduced and iron hotspots being more oxidized ( Fig. 4 ). Third, based on comparison of our specimens to XANES spectra of standard materials using linear combination fitting, incorporated iron was best accounted for by ~50 (±14)% each of iron (II) acetate and the iron (III) oxide goethite ( Fig. 3 ), suggesting the presence of a significant fraction of reduced organic iron. On the other hand, iron hotspots were best fitted by minerals containing oxidized iron (that is, ~66 (±24)% haematite and 34 (±24)% goethite on average) (Fig. 3 ). Finally, the reduced oxidation state of iron colocalizing with silicon supports the conclusion that iron is structurally incorporated and is, therefore, a natural component of biogenic silica, as any reduced iron unprotected from the ambient surface seawater would rapidly oxidize. The range of iron oxidation states observed in structurally incorporated iron might reflect gradual oxidation of iron over time, or a naturally mixed redox composition. 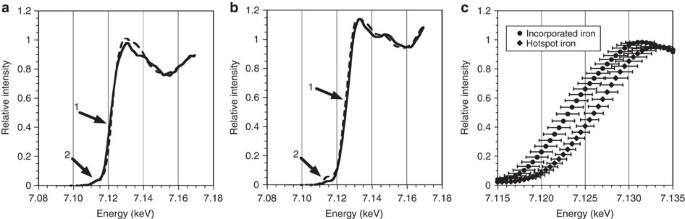Figure 3: Iron XANES spectra. Iron XANES spectra were collected from regions of iron incorporated into silica and iron hotspots identified in single specimens (for example,Fig. 1). A typical XANES spectrum collected from a single region of incorporated iron (a, solid line) exhibits a lower K-edge (1) and a lower pre-edge centroid position (2) than a typical single iron hotspot (b, solid line), indicating a difference in oxidation. Similarly, individual XANES spectra were fit using various proportions of standard iron phases (a,b, dashed lines). Taking into account the fit of all XANES spectra, incorporated iron was best accounted for on average by 49.9 (±14.0)% iron (II) acetate and 50.1 (±14.0)% of the iron (III) oxide goethite. On the other hand, iron hotspots were best accounted for on average by the oxidized iron minerals haematite (65.5 (±24.0)%) and geothite (34.5 (±24.0)%). Single XANES spectra for each iron pool were averaged (c). The difference in K-edge position between these average spectra (2.8±0.3 eV) is also consistent with incorporated iron being reduced and hotspot iron being oxidized. Error bars increpresent s.d. across a sample size of 7 and 19 spectra for incorporated and hotspot iron, respectively. All plots were generated from untreated samples (that is, no peroxide or acid treatment). Figure 3: Iron XANES spectra. Iron XANES spectra were collected from regions of iron incorporated into silica and iron hotspots identified in single specimens (for example, Fig. 1 ). A typical XANES spectrum collected from a single region of incorporated iron ( a , solid line) exhibits a lower K-edge (1) and a lower pre-edge centroid position (2) than a typical single iron hotspot ( b , solid line), indicating a difference in oxidation. Similarly, individual XANES spectra were fit using various proportions of standard iron phases ( a , b , dashed lines). Taking into account the fit of all XANES spectra, incorporated iron was best accounted for on average by 49.9 (±14.0)% iron (II) acetate and 50.1 (±14.0)% of the iron (III) oxide goethite. On the other hand, iron hotspots were best accounted for on average by the oxidized iron minerals haematite (65.5 (±24.0)%) and geothite (34.5 (±24.0)%). Single XANES spectra for each iron pool were averaged ( c ). The difference in K-edge position between these average spectra (2.8±0.3 eV) is also consistent with incorporated iron being reduced and hotspot iron being oxidized. Error bars in c represent s.d. across a sample size of 7 and 19 spectra for incorporated and hotspot iron, respectively. All plots were generated from untreated samples (that is, no peroxide or acid treatment). 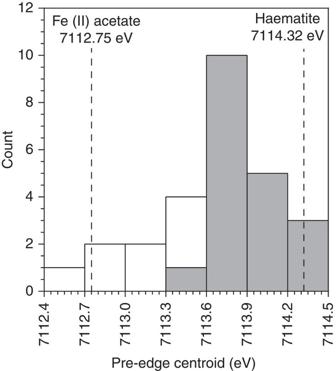Figure 4: Pre-edge centroid positions of iron XANES spectra. The distribution of pre-edge centroid positions among spectra collected from iron incorporated into silica (white bars) and micron-sized iron hotspots (grey bars) indicate a continuum of iron oxidation states, with incorporated iron clustering towards a more reduced state (for example, iron (II) acetate) and hotspot iron trending towards a more oxidized state (for example, the iron (III) mineral haematite). All plots were generated from untreated samples (that is, no peroxide or acid treatment). Full size image Figure 4: Pre-edge centroid positions of iron XANES spectra. The distribution of pre-edge centroid positions among spectra collected from iron incorporated into silica (white bars) and micron-sized iron hotspots (grey bars) indicate a continuum of iron oxidation states, with incorporated iron clustering towards a more reduced state (for example, iron (II) acetate) and hotspot iron trending towards a more oxidized state (for example, the iron (III) mineral haematite). All plots were generated from untreated samples (that is, no peroxide or acid treatment). Full size image Iron hotspots have been observed in other studies of Antarctic phytoplankton [13] , which, in addition to their presence in the current study, suggests they are a natural component of the particulate iron pool. The occasional spatial co-occurrence of hotspot iron with biogenic silica was likely coincidental, as iron hotspots were found both in association with biogenic silica and as isolated particles ( Fig. 1 ). Because of this random association, hotspots were systematically excluded from the calculation of iron-to-silicon ratios in biogenic silica. Iron-to-silicon ratios The ratio of iron to silicon in biogenic silica was determined for individual specimens using the per-area content of elements revealed in XRF micrographs, such as those presented in Fig. 1 . Ratios of iron to silicon in biogenic silica differed according to our method of chemical washing (untreated, acid-washed and peroxide-washed) ( Fig. 5 ). We focus on the group of specimens that were acid-washed because this treatment yielded the lowest and, therefore, most conservative estimate of iron in biogenic silica. Acid-washed biogenic silica specimens represented a variety of organisms, including silicoflagellates and diatoms of the genera Fragilariopsis and Corethron . Iron-to-silicon ratios in this group ranged from 14.8 to 493.3 μmol mol −1 , with a median value of 44.6 μmol mol −1 ( Fig. 5 ). 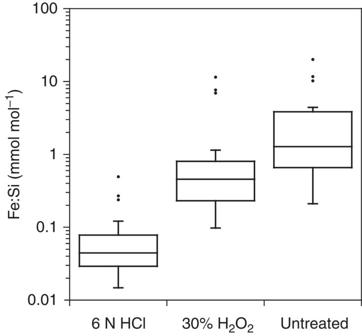Figure 5: Ratios of iron to silicon in biogenic silica. Silica specimens were examined untreated or after soaking in trace metal grade 6 N hydrochloric acid (HCl) or trace metal grade 30% hydrogen peroxide (H2O2) for 23 h. Middle quartiles of each sample group are defined by boxes. Median iron-to-silicon (Fe:Si) ratios (horizontal lines) of biogenic silica that was untreated, treated with H2O2and treated with HCl were 1.278, 0.458 and 0.045 mmol mol−1, respectively. The median across all groups was 0.328 mmol mol−1. Whiskers represent the sample range, excluding outliers. Outliers are at least 1.5 times greater or less than the upper or lower quartile, respectively. Sample sizes of the untreated, peroxide and acid-washed specimens are 17, 26 and 23, respectively. Figure 5: Ratios of iron to silicon in biogenic silica. Silica specimens were examined untreated or after soaking in trace metal grade 6 N hydrochloric acid (HCl) or trace metal grade 30% hydrogen peroxide (H 2 O 2 ) for 23 h. Middle quartiles of each sample group are defined by boxes. Median iron-to-silicon (Fe:Si) ratios (horizontal lines) of biogenic silica that was untreated, treated with H 2 O 2 and treated with HCl were 1.278, 0.458 and 0.045 mmol mol −1 , respectively. The median across all groups was 0.328 mmol mol −1 . Whiskers represent the sample range, excluding outliers. Outliers are at least 1.5 times greater or less than the upper or lower quartile, respectively. Sample sizes of the untreated, peroxide and acid-washed specimens are 17, 26 and 23, respectively. Full size image Our measurements of iron and silicon content in biogenic silica agree well with previous results obtained with different methods (iron-to-silicon ratios of 16 to >50 μmol mol −1 for cultivated isolates of the marine diatom Thalassiosira pseudonana ) [5] . Previous studies indicate that the incorporation of iron into silica is biologically controlled [5] , yet the potential physiological function of iron incorporation remains unknown. Certain evidence suggests a role for iron in biosilicification. For example, iron availability influences silicification kinetics independently of growth [16] , and correlations in the expression of silicification and iron uptake genes have been observed [17] . Depending on the stability of silica in the deep ocean and compositional changes to biogenic silica during diagenesis, a significant fraction of iron incorporated into silica may be sequestered from surface waters. For example, the net sinking flux of silica from Ross Sea surface waters is ~1 mol m −2 per year [18] , [19] ( Supplementary Information ). Using the conservative iron-to-silicon ratio for acid-washed biogenic silica specimens calculated above, we estimate that the loss of iron from surface waters through the vertical flux of silica in the Ross Sea is 45 μmol m −2 per year. This removal is at least approximately four times higher than the input of iron through snow melt and dust deposition (1.1–12.5 μmol m −2 per year) [20] , [21] , the principal sources of bioavailable iron in this area [20] , [22] . As a consequence of long-term diagenetic processes, silica burial in Ross Sea sediments is ~0.25 mol m −2 per year [19] . This accumulation could lead to a permanent iron burial flux of 11 μmol m −2 per year, which is comparable to iron input fluxes noted above. We calculate that the sequestration of iron could be up to 28 times greater if the iron-to-silicon ratio of untreated siliceous phytoplankton is more indicative of burial conditions, or if biogenic iron associated with non-siliceous cell structures is significant [23] . As biogenic iron associated with non-siliceous cell structures is most likely remineralized at a faster rate than structurally incorporated iron, this pool likely contributes little to the loss of iron from surface waters unlike the flux of recalcitrant, incorporated iron, which we propose. Furthermore, the magnitudes of our estimates clearly indicate that iron sequestration through the removal of silica from surface waters has a strong potential to control the bioavailable pool of iron in the Ross Sea, and perhaps other ocean areas, over a range of timescales. Iron removal through incorporation into silica may be particularly important in the pelagic Southern Ocean, where iron often limits growth [24] and the sedimentation and burial of biogenic silica are especially high [1] . The long-term burial rate of silica in Southern Ocean sediments is approximately twice that in the Ross Sea [1] . Using similar assumptions as above, we estimate that the long-term iron removal through incorporation into silica is ~23 μmol m −2 per year. Although a higher level of biologically relevant iron sequestration may occur over shorter timescales through the export of silica below the mixed layer, the major inputs of bioavailable iron to the Southern Ocean through lateral advection (for example, 9–45 μmol m −2 per year) [25] and atmospheric deposition (for example, 1–30 μmol m −2 per year) [25] , [26] , [27] are comparable to this long-term sink. As in the Ross Sea, the removal of iron through silica burial in the Southern Ocean may be a profound factor controlling the bioavailable pool of iron and, therefore, the primary productivity. Indeed, our estimated long-term iron removal flux through silica burial can account for ~30–90% of the export of particulate iron from surface waters in several typical systems of the Southern Ocean [25] . Similarly, removal of iron through incorporation into silica may also have a substantial role in the high-nutrient, low-chlorophyll equatorial Pacific, where iron burial is integrally, yet enigmatically, coupled to silica deposition [28] . Iron fertilization typically stimulates abundant diatom growth [12] , [29] , [30] , [31] . Therefore, incorporation of iron into diatom-derived silica may be a large sink of iron added during anthropogenic fertilization over timescales consistent with biological carbon fixation. This loss would be especially important if silica is rapidly exported below the mixed layer, as is the case in recently published results from the EIFEX iron fertilization experiment [12] . Moreover, stimulation of diatom growth by iron fertilization may result in more rapid iron removal than if non-silicifying organisms were stimulated. Enhanced iron removal through incorporation into biogenic silica may potentially shift microbial communities towards organisms with relatively lower iron requirements. For example, the non-silica-bearing prymnesiophyte, Phaeocystis antarctica , which can also dominate coastal Antarctic phytoplankton communities [6] , may be a poor competitor against diatoms under low iron availability [9] . Enhanced iron removal by incorporation into silica may therefore lead to longer periods of diatom dominance during the growing season, although this shift would be eventually counteracted when another nutrient became limiting, such as silicon or light. However, as P. antarctica assimilates carbon dioxide more efficiently than diatoms [6] , shifts towards diatom-dominated phytoplankton communities may dampen the intended outcome of iron fertilization (that is, enhanced carbon uptake). Thus, reduction of anthropogenic or natural iron pools through incorporation of iron into biogenic silica followed by vertical transport below the mixed layer may weaken the carbon dioxide uptake capacity of marine surface waters not only by imposing iron limitation on the existing photosynthetic community but also by altering microbial community composition in favour of organisms with less-efficient carbon assimilation. Sampling locations Samples were collected from polynya waters (76° 50.48′S 156° 22.93′W, depth ~500 m) and sea ice (74° 26.27′S 150° 38.50′W, depth~3,500 m) during the 2008/2009 austral summer expedition of the icebreaker Oden . Sample collection and preparation Polynya samples were collected using a plankton net (48 μm mesh). Sea ice was collected using a Kovacs Mark V fibreglass coring system (0.14 m diameter) with brand-new stainless steel cutting teeth. The sea‐ice core was sliced with a clean stainless steel saw into 10-cm horizons, transferred to acid‐washed plastic containers and diluted to 50% with filtered under-ice seawater to prevent salinity shock upon melt. The samples were slowly melted on a slow shaker table (dark; 15 °C) for ~24 h. Samples were stored in clean 15 ml polycarbonate tubes that had been rinsed multiple times with local seawater and were frozen (−20 °C) until further processing for trace metal analysis. To prepare samples for trace metal analysis, specimens were cleaned in trace metal grade 30% hydrogen peroxide (H 2 O 2 ) for 23 h or trace metal grade 6 N hydrochloric acid (HCl) for 23 h. The H 2 O 2 treatment targeted organic material on the surface of the plankton, and the HCl was used to remove organic coatings and loosely associated metals [14] . After each cleaning procedure, samples were washed twice in deionized water. The samples were mounted on gold transmission electron microscopy grids according to Twining et al. [13] , [23] and were allowed to dry. Grids were handled with Teflon-coated forceps. Synchrotron-based X-ray analyses X-ray analyses were performed on beamlines 2-ID-D and 2-ID-E at the Advanced Photon Source, Argonne National Laboratory. For XRF microscopy, the incident energy was 10 keV for beamline 2-ID-E and 7.2 keV for beamline 2-ID-D. Individual specimens were characterized for elemental content (atomic numbers from aluminium to iron) with a focused X-ray beam with a spot of size of ~200 × 200 nm for both beamlines. These beam spot sizes were smaller than the size of the two main features of interest: iron hotspots (~1 μm in diameter) and high iron areas of individual siliceous phytoplankton (>1 μm). Samples were mounted perpendicular to the beam. The thickness of a typical organism was 20–70 μm, whereas the depth of focus was at least 90 μm under all experimental configurations. For some samples, the beam was rastered over an individual specimen by taking steps at approximately the same resolution of the beam spot to create the highest resolution X-ray fluorescence map of the organism. Mapping at this resolution was time consuming, so it wasn’t done for every specimen. To maximize the number of specimens analysed in the allotted time, many maps were constructed rastering the beam in 1 μm steps using the spot size described above. This created a lower spatial resolution map, yet even at this lower resolution all relevant features were clearly discernable. Iron speciation was investigated with the focused beam at sub-500 nm spatial scales using XANES spectroscopy. XANES measurements were collected by scanning samples across a range of X-ray energies (7,090–7,170 eV in 0.5 eV steps, 0.5–10 s dwell time per step) and collecting the iron fluorescence signal at each step. The zone plate used for XANES measurements was 160 μm in diameter and the focal length was 64.4 mm at 7,130 eV. The sample was in focus at 7,130 eV. It is not expected that the focused beam size variation that typically occurs during XANES scans will alter the results in any substantial way ( Supplementary Information ). A range of dwell times were used, within practical limits, to maximize the number of fluorescence counts collected relative to the background. For regions with high iron concentration, several thousand iron counts could be obtained with a dwell time as low as 0.5 s. For lower iron areas, a 10-s dwell was sufficient to obtain XANES spectra. To address the possibility of systematic differences in pre-edge centroid position related to variations in count rate, a table of dwell times and the maximum counts for all samples presented in Fig. 4 is available in Supplementary Information ( Supplementary Table S1 ). In this table we have used the dwell and maximum count data to estimate the maximum count rate for each spectra. As one can see in Supplementary Table S1 , there is some overlap in hotspot and incorporated iron count rates, yet these samples have very different pre-edge centroid positions. In addition, within a class of specimen, a high count rate did not always correspond to a more oxidized pre-edge centroid position. Both these observations suggest that count rates do not confound estimation of oxidation state from spectral data. Following the typical procedure of XANES studies, data were normalized to account for small variations in beam intensity that can occur during data collection. Such variations in beam intensity were monitored with an ion chamber mounted upstream of the sample. After normalizing to the upstream ion chamber, the data was also processed using ten iterations of a three-point smoothing algorithm built into the software Athena [32] . Finally, the data for an individual XANES spectrum were normalized to create a relative intensity value of ~1 for post edge area of the spectra [32] as seen in Fig. 3 . Raw data for the spectra presented in Fig. 3 are presented in Supplementary Fig. S1 . The same features can be seen in the raw data as that seen in the normalized and smoothed data presented in Fig. 3 . Both XRF mapping and XANES spectra were collected under a helium environment using an energy dispersive silicon drift detector (Vortex EM, with a 50-mm 2 sensitive area with a 12.5-μm Be window; SII NanoTechnology, Northridge CA, USA). Full fluorescence spectra were fit with modified Gaussian curves to obtain counts relevant for the mapping and spectral analyses. For XRF elemental maps, average per-area densities (in units of μg cm −2 ) were calibrated with the thin-film standards NBS-1832 and NBS-1833 from the National Bureau of Standards (Gaithersburg, MD). Data analysis Elemental content of individual specimens was determined from XRF elemental maps using MAPS software [33] . Total element concentrations were calculated for user-defined regions of interest, allowing iron hotspots to be systematically removed from calculations of incorporated iron. The pre-edge centroid of iron XANES spectra has been found to be reliable for determination of iron oxidation state [15] , [34] . Pre-edge centroid positions in iron XANES spectra were determined using procedures described in Oakes et al. [34] Briefly, the background absorption was modelled by interpolating a cubic spline equation through the data 1 eV before and after the pre-edge feature. Once the background was determined, it was subtracted from the raw data, which allowed the shape and position of the pre-edge centroid to be better defined. A Gaussian equation was then fit to the background-corrected pre-edge feature using a peak fitting function in Igor software (version 6.1). Iron oxidation state was determined using a previously determined relation between pre-edge centroid position and iron oxidation state [34] . Linear combination fitting was performed for XANES spectra with the software Athena [32] , using standards collected on the same beamline used for sample analysis [34] . Data for iron standards is tabulated in Supplementary Data 1 . Athena uses a non-linear, least-squares minimization approach to optimize the linear combination results. The result with the lowest aggregate intensity difference to the sample spectrum (or R-factor) is considered the best fit [32] , [35] . Because of the limitation of available standards, particular iron species were chosen to represent a broader class of compounds ( Supplementary Information ). For example, iron (II) acetate was used to represent a simple organic-associated iron (II) compound. A standard was considered to have a substantial contribution if it accounted for more than 10% of a linear combination fit. How to cite this article: Ingall, E. D. et al. Role of biogenic silica in the removal of iron from the Antarctic seas. Nat. Commun. 4:1981 doi: 10.1038/ncomms2981 (2013).